CRISPR/Cas9-mediated gene targeting inArabidopsisusing sequential transformation Homologous recombination-based gene targeting is a powerful tool for precise genome modification and has been widely used in organisms ranging from yeast to higher organisms such as Drosophila and mouse. However, gene targeting in higher plants, including the most widely used model plant Arabidopsis thaliana , remains challenging. Here we report a sequential transformation method for gene targeting in Arabidopsis . We find that parental lines expressing the bacterial endonuclease Cas9 from the egg cell- and early embryo-specific DD45 gene promoter can improve the frequency of single-guide RNA-targeted gene knock-ins and sequence replacements via homologous recombination at several endogenous sites in the Arabidopsis genome. These heritable gene targeting can be identified by regular PCR. Our approach enables routine and fine manipulation of the Arabidopsis genome. Precise genome modification such as DNA knock-in and gene replacement (i.e., gene targeting) via homologous recombination is a powerful tool that is widely applied for research in many organisms, including Drosophila and animals [1] , [2] , [3] . However, gene targeting (GT) is still very challenging in higher plant species, because of low efficiency of homologous recombination [4] . Engineered sequence-specific nucleases such as zinc finger nucleases (ZFNs), transcription activator-like effector nucleases (TALENs) and clustered regularly interspaced short palindromic repeats (CRISPR)/CRISPR-associated protein 9 (Cas9) have been used to generate site-specific double stranded breaks (DSBs) for genome editing in numerous organisms [1] , [5] , [6] , [7] . Repair of these DSBs via error-prone non-homologous end-joining (NHEJ) leads to random mutations, whereas error-free homology-directed repair (HDR) creates precise sequence changes when a homologous DNA substrate is provided. A goal of genome editing is to achieve heritable GT, defined as the precise insertion or replacement of sequence at any genomic locus of interest in germline cells. However, HDR-mediated GT at endogenous genes is extremely inefficient in higher plants, preventing its widespread application [4] . The first GT in plants was demonstrated at a kanamycin resistance gene in tobacco, with a frequency ranging from 10 −3 to 10 −6 (refs. [8] , [9] ). A higher efficiency method using positive−negative selection was later developed in rice [10] ; however, this complicated strategy has been used to modify only several genes in rice [11] and has not been successfully applied to other plants, including Arabidopsis [12] , [13] and tobacco [14] . Sequence-specific nucleases can increase the efficiency of GT [1] , [15] , [16] , and CRISPR/Cas9-assisted HDR has been used for GT in various model systems, including human stem cells [15] . The introduction of DSBs also increased the frequency of HDR in plants [17] , [18] , and recent publications report using sequence-specific nucleases for HDR-mediated GT in Arabidopsis [19] , [20] , [21] , [22] , [23] , [24] , tobacco [25] , [26] , [27] , [28] , [29] , [30] , soybean [31] , tomato [32] , [33] , rice [34] , [35] , [36] , [37] , [38] , [39] , [40] , [41] , maize [42] , [43] , [44] , [45] , [46] , wheat [47] , [48] , potato [49] , barley [50] , flax [51] , and cotton [52] . Nevertheless, these GT events mostly relied on selection for antibiotic or herbicide resistance genes at the targeted loci to improve efficiency. The few GT events that did not rely on selection markers displayed extremely low frequencies [24] , [31] , [43] , thus limiting the usefulness of these methods. Here, we describe a simple method for seamless GT in Arabidopsis , including in-frame gene knock-ins and amino acid substitutions. We demonstrate the utility of our method by targeting the endogenous DNA glycosylase genes ROS1 and DME in Arabidopsis . Inefficient GT by an all-in-one strategy To achieve efficient GT in Arabidopsis , we first designed an “all-in-one” T-DNA construct that contains: (i) Cas9 driven by the CaMV 35S promoter (35Spro::Cas9), (ii) an sgRNA driven by the AtU6 promoter, that targets a site near the stop codon of ROS1 , and (iii) a donor DNA fragment for in-frame GFP knock-in (Supplementary Fig. 1a ). We screened T1 plants by PCR (e.g. Supplementary Fig. 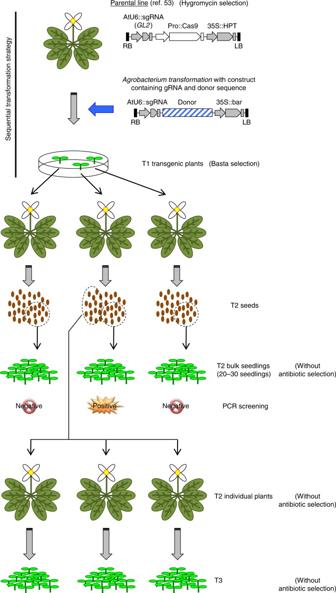Fig. 1 Outline of the sequential transformation strategy for gene targeting and screening procedure. HDR donor constructs containing a selection marker and sgRNAs targeting genes of interest were transformed into parental lines, which were already transgenic for an incidentalGL2-targeting sgRNA and, importantly, for Cas9 driven by a specific promoter. T1 transgenic lines were selected with Basta, and T2 seedlings were obtained and analyzed in bulk. The positive lines were used for further experiments with individual T2 plants. Portions of the images were obtained from the Microsoft PowerPoint clip art data base 1b ), and identified 2/30 with a positive GT signal (Supplementary Table 1 ). In contrast, a control construct without an sgRNA did not yield any T1 plants with a positive GT signal (Supplementary Table 1 ). Neither of the T1-positive plants gave rise to T2 progenies with a positive GT signal, although bulk screening of 18 remaining T2 lines identified a positive GT signal (Supplementary Table 1 ). Southern blot analysis of individual plants from this PCR-positive T2 population failed to detect any GT-positive plants (Supplementary Fig. 1b ), suggesting that the GT-positive PCR signal may have come from a small number of somatic cells. Thus, this method did not generate heritable GT. A similar all-in-one construct also failed to generate heritable in-frame ROS1 - Luc knock-ins (Supplementary Table 1 ). The expression of Cas9 under germline-specific promoters was recently shown to increase the efficiency of CRISPR/Cas9-mediated gene editing in Arabidopsis [53] , [54] , [55] . We hypothesized that driving Cas9 expression from a germline-specific promoter instead of the CaMV 35S promoter might increase the frequency of heritable GT. We tested the following promoters: the egg cell- and early embryo-specific promoter DD45 [53] , [54] , [56] , the pollen-specific promoter Lat52 [53] , and the shoot apical meristem-active promoters YAO [55] and CDC45 [57] . We generated all-in-one constructs for GFP knock-in into the GLABRA2 ( GL2 ) locus, utilizing these promoters to drive Cas9 expression and an sgRNA known to efficiently generate site-specific DSB in GL2 [53] (Supplementary Fig. 1c ). Although we observed high frequencies of GT-positive PCR signals with some of these all-in-one constructs, we did not identify any heritable GT lines (Supplementary Fig. 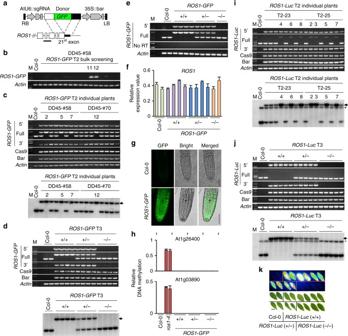Fig. 2 GFPintegration into the endogenousROS1locus by gene targeting.aSchematics showing HDR donor transgene construct (top) and part of the targetedROS1locus (bottom). The horizontal line indicates the position of a probe for Southern blot hybridization.bPCR screening of T2 bulk samples (see Supplementary Figure2). Primers for the 5′ part ofROS1-GFPwere used (see Supplementary Figure2).c,dGenotyping PCR and Southern blotting of a subset of individual T2 (c) and T3 plants (d) ofROS1-GFP, respectively. The eight plants in the DD45-#58 background were selected from populations 11 and 12 in (b). Arrow indicates the band ofROS1-GFPfrom gene targeting.eRT-PCR andfqRT-PCR on the same T3 plants as in (d). The error bars indicatePvalues of Student’sttest (n= 4). See Supplementary Figure2.gDetection of GFP fluorescence. Scale bar, 50 µm.hqChop-PCR at the At1g26400 and At1g03890 loci. Theros1-4mutant was used as a positive control. The error bars indicatePvalues of Student’sttest (n= 4).i,jGenotyping PCR and Southern blotting for individual T2 lines (i) and T3 plants (j) ofROS1-Luc, respectively. Arrow indicates the band ofROS1-Lucfrom gene targeting, and the asterisk denotes non-specific cross-hybridization band.kLuminescence in T3ROS1-Lucleaves. Scale bar, 1 cm. All PCR primers are as depicted in Supplementary Figure2b, cand Supplementary Table4 1d–i , Supplementary Table 2 ). Sequencing of the PCR products indicated that precise GT events occurred, but they likely represent minor events in some somatic cells. Thus, although expression of Cas9 under these specific promoters might improve GT efficiency in some somatic tissues, it did not lead to heritable GT. Knock-in into the ROS1 locus by sequential transformation Next, we used a “sequential transformation method” to evaluate GT efficiency [35] , [41] in parental Arabidopsis plants that already express Cas9 from a germline-specific (DD45, Lat52, YAO or CDC45) promoter (Fig. 1 ). These parental Cas9 lines also express a GL2 -targeting sgRNA from the AtU6 promoter. We used the two highest efficiency CRISPR/Cas9 lines, which were screened from 32 to 36 independent T1 lines based on the mutation rates at the GL2 locus, for each specific promoter [53] . We used these Cas9-expressing plants as parental lines for new transformations with a construct containing: (i) HDR donor sequence, (ii) sgRNA targeting a genomic locus of interest, (iii) a selectable marker for plants that are positive for the donor construct (Figs. 1 , 2a ). The new transformation T1 transgenic plants were selected using the Basta resistance gene. These T1 plants express Cas9 and a specific sgRNA, and contain a specific HDR donor sequence. T1 seeds were harvested and germinated without selection on MS plates; 20−30 of the resulting T2 seedlings were subsequently pooled together, and GT events were analyzed by PCR in bulk. Further, another batch of T2 plants from the bulk positive lines were investigated as individual plants (Fig. 1 ). Fig. 1 Outline of the sequential transformation strategy for gene targeting and screening procedure. HDR donor constructs containing a selection marker and sgRNAs targeting genes of interest were transformed into parental lines, which were already transgenic for an incidental GL2 -targeting sgRNA and, importantly, for Cas9 driven by a specific promoter. T1 transgenic lines were selected with Basta, and T2 seedlings were obtained and analyzed in bulk. The positive lines were used for further experiments with individual T2 plants. Portions of the images were obtained from the Microsoft PowerPoint clip art data base Full size image Fig. 2 GFP integration into the endogenous ROS1 locus by gene targeting. a Schematics showing HDR donor transgene construct (top) and part of the targeted ROS1 locus (bottom). The horizontal line indicates the position of a probe for Southern blot hybridization. b PCR screening of T2 bulk samples (see Supplementary Figure 2 ). Primers for the 5′ part of ROS1 - GFP were used (see Supplementary Figure 2 ). c , d Genotyping PCR and Southern blotting of a subset of individual T2 ( c ) and T3 plants ( d ) of ROS1 - GFP , respectively. The eight plants in the DD45-#58 background were selected from populations 11 and 12 in ( b ). Arrow indicates the band of ROS1 - GFP from gene targeting. e RT-PCR and f qRT-PCR on the same T3 plants as in ( d ). The error bars indicate P values of Student’s t test ( n = 4). See Supplementary Figure 2 . g Detection of GFP fluorescence. Scale bar, 50 µm. h qChop-PCR at the At1g26400 and At1g03890 loci. The ros1 - 4 mutant was used as a positive control. The error bars indicate P values of Student’s t test ( n = 4). i , j Genotyping PCR and Southern blotting for individual T2 lines ( i ) and T3 plants ( j ) of ROS1 - Luc , respectively. Arrow indicates the band of ROS1 - Luc from gene targeting, and the asterisk denotes non-specific cross-hybridization band. k Luminescence in T3 ROS1 - Luc leaves. Scale bar, 1 cm. All PCR primers are as depicted in Supplementary Figure 2b, c and Supplementary Table 4 Full size image Transformation of a construct containing ROS1 -targeting sgRNA and ROS1 - GFP donor sequence into DD45pro::Cas9 lines #58 and #70, but not other promoter::Cas9 lines, gave rise to Southern blot- and PCR-positive GT signals (Fig. 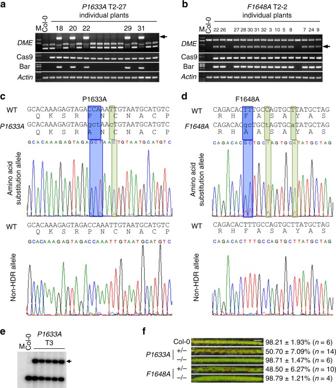Fig. 4 Single amino acid substitution at the endogenousDMElocus by gene targeting.a,bGenotyping of T2 individual plants forP1633AandF1648A, respectively. Arrows indicate the specific sequence substitution as detected by PCR and restriction enzyme digestion. PCR primers are as depicted in Supplementary Figure 6aand Supplementary Table4. Detailed information is described in Supplementary Figure6.c,dSequence confirmation of theP1633AandF1648Asubstitutions, respectively, in individual T2 plants. Blue highlights indicate amino acid substitution, green highlights indicate silent mutations. The sequence chromatograms are taken from FinchTV.eSouthern blotting. TheP1633Asubstitutions were confirmed by Southern blotting in heterozygous T3 plants. The arrow indicates the band caused by specific base substitution.fAnalysis of seed abortion. Seeds from Col-0, heterozygous GT (+/−), and non-GT (−/−)P1633AandF1648AT3 plants were analyzed. Scale bar, 1 mm 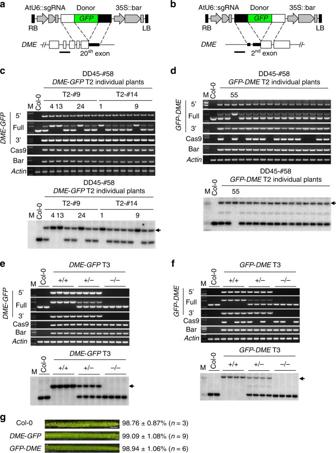2a−c , Table 1 , Supplementary Fig. Fig. 3 GFPknock-in into the endogenousDMElocus by gene targeting.a,bSchematics showing HDR donor transgene constructs and part of the targetedDMElocus forDME-GFPandGFP-DMEknock-in, respectively. The horizontal lines indicate the positions of probes for Southern blotting.c−fGenotyping PCR and Southern blotting for individual T2 lines (b) and T3 plants (e) ofDME-GFP, respectively. Arrow indicates the band ofDME-GFPfrom gene targeting (see Supplementary Figure3). Genotyping PCR and Southern blotting for individual T2 lines (d) and T3 plants (f) ofGFP-DME, respectively. Arrow indicates the band ofGFP-DMEfrom gene targeting (see Supplementary Figure3).gAnalysis of seed abortion. Seeds from Col-0, homozygousDME-GFP, andGFP-DMEknock-in T3 plants were analyzed. Scale bar, 1 mm. All PCR primers are as depicted in Supplementary Figure3and Supplementary Table4 2 , Supplementary Table 3 ). Six out of 11 tested plants from two T2 populations in the DD45-#58 background were homozygous ROS1 - GFP GT lines based on Southern blot analysis, and 2 of 12 tested plants from another two T2 populations in the DD45-#70 background were homozygous (Table 1 ; e.g. Fig. 2c ). Sanger sequencing confirmed that there were no mutations in the 5′ and 3′ homology arms and their border regions, and that GFP integration downstream of the ROS1 gene was in-frame (Supplementary Figs. 4 a and 5a ). We examined the progenies of a heterozygous T2 GT plant and found that the integrated ROS1 - GFP segregated in T3 (Fig. 2d ). We analyzed mRNA expression in these T3 plant samples by RT-PCR and qRT-PCR, and observed comparable expression of the ROS1 - GFP knock-in with endogenous ROS1 (Fig. 2e, f ). Further, the root tissues of homozygous T3 ROS1 - GFP plants displayed GFP fluorescence (Fig. 2g ). To determine whether the ROS1 - GFP knock-in retained ROS1 function, we assessed the DNA methylation level of two genomic loci known to become hypermethylated in loss-of-function ros1 mutant plants by quantitative Chop-PCR (Fig. 2h ) [58] . Homozygous T3 ROS1-GFP knock-in plants did not display hypermethylation at these loci, suggesting that the in-frame integration of GFP did not interfere with ROS1 function, and that the ROS1 - GFP was functional. Thus, our sequential transformation method efficiently generates precise and heritable GT. Table 1 Knock-in GT efficiencies for the ROS1 and DME loci Full size table Next we tested whether a fragment longer than GFP could be integrated at the ROS1 locus. We used the same sgRNA and homology arms to make a donor construct that contained firefly luciferase ( Luc : 1653 bp) instead of GFP (720 bp), and transformed the construct into parental CRISPR/Cas9 lines. Two positive GT lines were identified in T2 bulk screening by PCR, and precise knock-in was confirmed in individual T2 and T3 plants (Table 1 , Figs. 1 , 2i, j ). These true GT-positive (PCR and Southern blotting positive in individual T2 plants) ROS1 - Luc lines were all from the DD45pro::Cas9 background (Table 1 , Supplementary Table 3 ). The leaves of homozygous and heterozygous ROS1 - Luc T3 plants displayed luminescence signals, unlike those from control plants without GT (Fig. 2k ). Thus, a fragment as large as 1.6 kb can be stably integrated into a genomic locus using our sequential transformation GT strategy. Knock-in into the DME locus Next, to investigate the broad utility of our GT method, we attempted to generate in-frame GFP knock-ins at the 5′ end and the 3′ end of DME (At5g04560), a DNA glycosylase gene on a different chromosome than ROS1 in Arabidopsis . We designed specific sgRNAs and donor constructs for a 3′ in-frame fusion ( DME - GFP ) and 5′ in-frame fusion ( GFP - DME ) (Fig. 3a, b , Supplementary Fig. 3 ). The sgRNA used to generate GFP-DME also targets the 3′ homology region of the donor construct, so we introduced silent mutations within the 3′ donor sequence of GFP - DME to prevent sgRNA binding, DSB and mutations following precise knock-in (Supplementary Fig. 3b ). Fig. 3 GFP knock-in into the endogenous DME locus by gene targeting. a , b Schematics showing HDR donor transgene constructs and part of the targeted DME locus for DME - GFP and GFP - DME knock-in, respectively. The horizontal lines indicate the positions of probes for Southern blotting. c−f Genotyping PCR and Southern blotting for individual T2 lines ( b ) and T3 plants ( e ) of DME - GFP , respectively. Arrow indicates the band of DME - GFP from gene targeting (see Supplementary Figure 3 ). Genotyping PCR and Southern blotting for individual T2 lines ( d ) and T3 plants ( f ) of GFP - DME , respectively. Arrow indicates the band of GFP - DME from gene targeting (see Supplementary Figure 3 ). g Analysis of seed abortion. Seeds from Col-0, homozygous DME - GFP , and GFP - DME knock-in T3 plants were analyzed. Scale bar, 1 mm. All PCR primers are as depicted in Supplementary Figure 3 and Supplementary Table 4 Full size image These T-DNA constructs were transformed into the parental Lat52, YAO, CDC45, and DD45 promoter-driven CRISPR/Cas9 lines. Although some GT signals were detected by PCR in the T1 and T2 plants from the Lat52, YAO and CDC45 parental lines, they were not heritable GT events, given that positive signals were not detected by Southern blotting or in some cases even by PCR in individual T2 plants (Supplementary Table 3 ). In contrast, true GT-positive (PCR and Southern blotting positive in individual T2 plants) signals were detected for DME - GFP from 2 out of 22 T2 populations (9.1%) in the DD45-#58 parental line (Table 1 ). Further, two positive GT signals were detected for GFP - DME from 24 T2 populations (8.3%), from each of the DD45-#58 and DD45-#70 parental lines (Table 1 ). Analysis of individual T2 plants revealed homozygous and heterozygous plants for both DME - GFP and GFP - DME fusions (Fig. 3c, d , Supplementary Fig. 3 ). The heterozygous T2 plants segregated in T3 (Fig. 3e, f , Supplementary Fig. 3 ). These in-frame GFP knock-ins at the 5′ and 3′ ends of DME were confirmed by sequencing the PCR products (Supplementary Figs. 4b , c, 5b, c ). Homozygous and heterozygous DME - GFP and GFP - DME plants did not show any developmental or growth defects, suggesting that the gene-targeted DME is functional, since dme loss-of-function mutants show maternal lethality [59] . To further confirm that the DME - GFP and GFP - DME in-frame fusion proteins are functional, we examined the seed abortion ratios of homozygous DME - GFP and GFP - DME T3 plants, and found that they were comparable with that of wild-type Col-0 plants (Fig. 3g ). Thus, the DME - GFP and GFP - DME in-frame fusions are functional. Sequence replacement at the DME locus An important goal of GT is the fine manipulation of endogenous genes by gene replacement. To test the feasibility of gene replacement, we attempted to substitute an amino acid within a conserved motif of DME (Supplementary Fig. 6 ). The Fe-S motif is highly conserved in the family of 5-methylcytosine DNA glycosylases, and is required for 5-methylcytosine DNA glycosylase activity of DME and ROS1 in vitro [60] , [61] . We generated mutated forms of a DME donor by changing a conserved proline to alanine (P1633A) and phenylalanine to alanine (F1648A). Silent mutations were also integrated at the PAM sequence to block additional DSBs, following the CORRECT method [15] (Supplementary Fig. 6 ). The two constructs containing the mutated DME donors and corresponding sgRNAs were transformed into YAO, CDC45, and DD45 promoter-driven CRISPR/Cas9 parental lines. We used a PCR-restriction enzyme assay to uncover amino acid substitution GT events. Heritable GT lines were obtained only in the DD45pro::Cas9 parental background (Fig. 4a, b , Table 2 , Supplementary Table 3 ). We sequenced the PCR amplicons from GT-positive T2 plants and found accurate amino acid substitutions, with no other mutations (Fig. 4c, d ). Southern blot analysis of several T3 plants revealed that they were all heterozygous for the amino acid substitution GT (Fig. 4e ). Thus, the amino acid substitution GT was stable and heritable. Fig. 4 Single amino acid substitution at the endogenous DME locus by gene targeting. a , b Genotyping of T2 individual plants for P1633A and F1648A , respectively. Arrows indicate the specific sequence substitution as detected by PCR and restriction enzyme digestion. PCR primers are as depicted in Supplementary Figure 6 a and Supplementary Table 4 . Detailed information is described in Supplementary Figure 6 . c , d Sequence confirmation of the P1633A and F1648A substitutions, respectively, in individual T2 plants. Blue highlights indicate amino acid substitution, green highlights indicate silent mutations. The sequence chromatograms are taken from FinchTV. e Southern blotting. The P1633A substitutions were confirmed by Southern blotting in heterozygous T3 plants. The arrow indicates the band caused by specific base substitution. f Analysis of seed abortion. Seeds from Col-0, heterozygous GT (+/−), and non-GT (−/−) P1633A and F1648A T3 plants were analyzed. Scale bar, 1 mm Full size image Table 2 Gene replacement efficiencies for the DME locus Full size table We did not obtain any homozygous P1633A and F1648A GT plants in T2 or T3 generations, likely due to the lethality of loss-of-function dme mutations [59] . Indeed, approximately 50% of the seeds of the P1633A and F1648A heterozygous T3 plants aborted, whereas no seed abortion was found in T3 plants without the amino acid substitution GT (Fig. 4f ). Thus, these two highly conserved amino acids within the Fe-S motif, P1633 and F1648, are essential for DME function in vivo. GT effect on DNA methylation ZFN-mediated GT of the endogenous locus PPOX in plants reportedly alters its epigenetic status [62] . We performed individual locus bisulfite sequencing to analyze whether DNA methylation is affected in two independent homozygous T4 ROS1 - GFP GT plants generated by our sequential GT strategy. We did not observe substantial changes in cytosine methylation in either the 5′ or 3′ homology arm regions (Supplementary Fig. 7 ), suggesting that our GT method did not affect the DNA methylation status of the targeted genomic locus. Using our new approach for efficient and heritable GT in Arabidopsis , we achieved precise knock-ins, generating ROS1 - GFP , ROS1 - Luc , DME - GFP , and GFP - DME fusions, as well as gene replacements, generating P1633A and F1648A amino acid substitutions in DME. Only parental plant lines expressing Cas9 under the egg cell- and early embryo-specific promoter DD45 gave rise to efficient and heritable GT, without any need for a selection marker at the targeted locus. The fact that only DD45 promoter-driven Cas9 lines yielded heritable GT suggests that HDR may be more efficient in egg cells and/or early embryos than in other germline tissues (e.g., pollen and shoot apical meristem). We propose that germline GT occurs immediately after transformation, when Agrobacteria enter the Cas9-expressing ovule [63] to deliver the T-DNA containing sgRNA and donor DNA. Efficient HDR may occur in the egg cell and/or very early embryo, perhaps before T-DNA integration. Alternatively, HDR and the resulting GT may occur during the reproductive stage of T1 plants, when the T-DNA is already stably integrated. Five GFP - DME heterozygous T2 plants showed segregation from the Cas9 transgene (Fig. 3e, f ), indicating that heritable knock-in occurred in T1 plants. The frequency of GT-positive plants in T2 populations ranged from 4/59 to 53/60 (Tables 1 and 2 ). The data are consistent with heritable GT events occurring in early embryos following the new transformation, in agreement with the strong activity of DD45 promoter in egg cells and early embryos [56] . All of the heritable GT events we observed were precise, without unexpected mutations or rearrangements at the target sites. The GT efficiency by our method was 5.3% for DME P1633A and was higher for other knock-ins or gene replacement (Tables 1 and 2 ). We analyzed T2 bulk DNA to determine whether the T-DNA copy numbers may contribute to efficient GT. Our results show that GT events were not related to T-DNA copy numbers of Cas9 or of the HDR donor transgene (Supplementary Fig. 8 ), suggesting that other unknown factors might be important. Additional research is required to understand and improve GT efficiency, and to apply this GT method to other plants including crops. Here we revealed heritable GT and simple PCR-based identification, without the need of any selection marker at the target locus. This approach enables routine GT in Arabidopsis . Using egg cell- and early embryo-specific promoters to drive the expression of Cas9 or other site-specific nucleases, in combination with strategies for the effective delivery of donor DNA (such as described in ref. [4] ), might lead to efficient GT technologies in other plants, including crop plants. Gene accession numbers ROS1 , At2g36490; DME , At5g04560; GL2 , At1g79840. Plant materials and growth condition The Arabidopsis thaliana accession Col-0 was used for all experiments. All plants were grown at 22 ˚C on half Murashige and Skoog (MS) medium with 1% sucrose or in soil with a 16 h light/8 h dark photoperiod. Parental T2 plants [53] were selected on the hygromycin (25 mg/L) containing MS plates for 10 days, then transplant in soil. The new transformation T1 lines were directly sowed in soil, and selected by three times Basta spray. Plasmid construction The optimized coding sequence of hSpCas9 (CRISPR/Cas9) plasmids for GL2 GT, which were already reported [53] , were constructed in pCambia1300. For all-in-one GT constructs, donor sequence was added to the published CRISPR/Cas9 constructs. For GT constructs for the sequential transformation strategy, AtU6 promoter-driven sgRNA and donor sequence were constructed in pCambia3301. All transformants were generated by the flower dipping method. DNA analysis Total DNA was extracted by the cethyltrimethyl ammonium bromide (CTAB) method from 10-day-old seedling for bulk analysis or 4- to 6-week-old for individual plant analysis. Extracted DNA was used for analysis of GT events by PCR and Southern blotting. Southern blotting was performed according to published protocols. Briefly, extracted DNA was digested overnight with chosen restriction enzymes, then separated on a 1.5% agarose gel, visualized by Image Lab Software and Gel Doc XR (BIO-RAD), and then transferred to nylon membrane (GE Healthcare). The probes were labeled with 32P-α-dCTP by using the Random primer DNA labeling kit (Takara). The hybridization signals were detected with a phosphor imager (Fuji). Un-cropped images of the most important Southern blots were supplied as Supplementary Fig. 10 . RNA analysis For RT- and qRT-PCR, total RNA was extracted form 10-day-old or 4-week-old plants by using RNeasy Plant mini kit (Qiagen), treated with Turbo DNA-free (Ambion), and reverse transcribed by TransScript II (TransGen Biotech) with oligo (dT) primer. Then 1 μL of RT product was used as template for expression analysis. The raw data of some of the qPCR analysis are shown in Supplemental Fig. 9. Detection of GFP fluorescence and Luc luminescence GFP signal was observed in the roots of 3-day-old seedlings by confocal microscopy (Leica TCS SP8). Bright field and GFP fluorescence images were merged using ImageJ. To determine firefly luciferase (Luc) reporter activity, 0.5 μM luciferin (Promega) in 0.01% Triton X-100 was sprayed onto 4-week-old mature leaves, followed by luminescence imaging using a high-performance CCD camera. DNA methylation analysis DNA methylation was analyzed by bisulfite sequencing. Total DNA was extracted using the CTAB method, and un-methylated cytosines were converted into uracil by using EZ DNA Methylation-Gold Kit (ZYMO RESEARCH). Genomic regions of interest were amplified by specific primers (Supplementary Table 4 ), then the amplicons were cloned into pMD-18 (Takara), and at least 27 independent colonies were sequenced. The sequence results were analyzed by Kismeth. Data availability The authors declare that all the data supporting the findings of this study are available within the paper and its supplementary information files. The data sets generated or analyzed during the current study are available from the corresponding author on reasonable request. We deposited our DD45::CRSIPR/Cas9 parental lines, DD45-#58 and DD45-#70, to the Arabidopsis Biological Resource Center (ABRC). The seeds were assigned the stock numbers CS69955 and CS69956, respectively. The two homozygous DD45::CRISPR/Cas9 parental lines could retain a high rate of GT when they are propagated to future generations with hygromycin selection.